Amplification of oxidative stress by a dual stimuli-responsive hybrid drug enhances cancer cell death Cancer cells, compared with normal cells, are under oxidative stress associated with the increased generation of reactive oxygen species (ROS) including H 2 O 2 and are also susceptible to further ROS insults. Cancer cells adapt to oxidative stress by upregulating antioxidant systems such as glutathione to counteract the damaging effects of ROS. Therefore, the elevation of oxidative stress preferentially in cancer cells by depleting glutathione or generating ROS is a logical therapeutic strategy for the development of anticancer drugs. Here we report a dual stimuli-responsive hybrid anticancer drug QCA, which can be activated by H 2 O 2 and acidic pH to release glutathione-scavenging quinone methide and ROS-generating cinnamaldehyde, respectively, in cancer cells. Quinone methide and cinnamaldehyde act in a synergistic manner to amplify oxidative stress, leading to preferential killing of cancer cells in vitro and in vivo . We therefore anticipate that QCA has promising potential as an anticancer therapeutic agent. Reactive oxygen species (ROS) are a group of highly reactive small molecules generated by all aerobic organisms and encompass H 2 O 2 , superoxide (O 2− ) and hydroxyl radical [1] , [2] . In particular, H 2 O 2 plays important roles in cell growth, proliferation and signalling pathway under physiological conditions [3] . Redox balance between oxidizing and reducing species within cells is important in the regulation of signalling pathway and is achieved by various enzymes such as superoxide dismutase, catalase and glutathione peroxidase [2] . However, overproduction of H 2 O 2 and other ROS causes oxidative stress, leading to cellular damages and subsequent functional decline of organ systems [4] , [5] . Therefore, it is crucial for normal cells to maintain ROS homeostasis to control the ROS level and overcome the potential toxicity of ROS [6] . Accumulating evidence has suggested that abnormal cancer cells are under oxidative stress associated with an increased production of ROS due to disrupted ROS homeostasis and cancer cells have also adapted to oxidative stress by activating antioxidant systems often through the upregulation of glutathione (GSH) [2] , [7] , [8] , [9] , [10] . Ironically, cancer cells are also known to utilize ROS to drive proliferation and other events required for tumour development [11] , [12] . However, the high level of ROS can cause cellular damage and apoptotic cell death, depending on the concentration and duration of ROS stress [13] . Cancer cells are also susceptible to further ROS insults induced by exogenous agents that weaken antioxidant defense or augment ROS generation to a level or the threshold above which cells cannot survive [14] , [15] , [16] . It was also postulated that cancer cells under oxidative stress are highly dependent on their antioxidant systems to counteract the damaging effects of ROS to maintain the ROS balance. Therefore, the difference in redox balance in normal and cancer cells would provide a biological cue for selective killing of malignant cancer cells [17] . Recently, there have been increasing efforts to develop a strategy to increase the level of ROS in cancer cells specifically, leading to ROS-mediated cancer cell death, which is named as ‘oxidation therapy’ [1] , [12] , [14] . One way of this anticancer therapy is to deliver ROS-generating agents to tumour tissues directly, such as arsenic trioxide (As 2 O 3 ) and glucose oxidase [17] . Another approach of oxidation therapy is to disrupt the redox balance in cancer cells by suppressing the antioxidant systems. There are several therapeutic agents that inhibit antioxidative enzyme systems and exert cytotoxicity to cancer cells, including L -buthionine-sulfoximine, β-phenylethyl isothiocyanate and zinc protoporphyrin [1] , [17] , [18] , [19] . These agents are known to induce non-severe ROS stress in normal cells because normal cells have a low level of basal ROS [11] , [16] . A newly discovered antioxidant inhibitor with anticancer activity is quinone methide (QM). QM was reported to rapidly alkylate GSH, one of the key antioxidant systems in cells and trigger apoptotic cell death [20] . Hulsman et al . [7] reported that the potent anticancer activity of nitric oxide-donating aspirin is attributed to QM, but not nitric oxide. Combined use of an ROS-generating agent with an inhibitor of ROS scavenging systems has been also reported to amplify oxidative stress and be effective in the treatment of advanced solid tumours in terms of both efficacy and selectivity [8] , [19] . Therefore, manipulating the ROS levels by redox modulation is a logical approach to selectively kill cancer cells without causing significant toxicity to normal cells and would have broad therapeutic applications for cancer treatment. In this study, we report a novel hybrid anticancer therapeutic agent that not only weakens the antioxidant defense systems but also elevates ROS production simultaneously, leading to massive ROS accumulation preferentially in cancer cells and subsequent ROS-mediated cell death ( Fig. 1 ). Cinnamaldehyde, a major component of cinnamon tree, has been known to induce intracellular ROS generation, leading to apoptotic cell death [21] , [22] . Cinnamaldehyde contains active Michael acceptor pharmacophore and is given the Generally Recognized as Safe status with approval for use in food in the United States [22] . Cinnamaldehyde has been reported to induce ROS generation mainly in the mitochondria and inhibit growth of human cancer cells, but minimal cytotoxicity to normal cells [21] , [23] , [24] . However, the clinical applications of cinnamaldehyde have been limited by its poor bioavailability (a short half-life in blood) due to rapid oxidation of aldehyde group and lower drug efficacy than common anticancer drugs [21] , [25] , [26] . 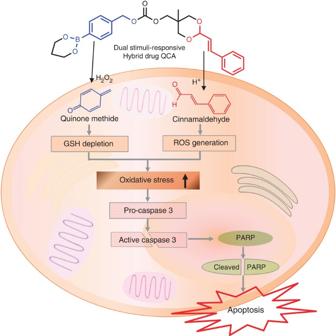Figure 1: A dual stimuli-responsive hybrid anticancer drug QCA. QCA is activated by H2O2and acidic pH and amplifies oxidative stress in cancer cells, leading to apoptotic cell death. Figure 1: A dual stimuli-responsive hybrid anticancer drug QCA. QCA is activated by H 2 O 2 and acidic pH and amplifies oxidative stress in cancer cells, leading to apoptotic cell death. Full size image To overcome these drawbacks, we developed QCA, [4-(1,3,2-dioxaborinan-2-yl)benzyl ((5-methyl-2-styryl-1,3-dioxan-5-yl)methyl) carbonate] as a novel hybrid anticancer prodrug by coupling a QM-generating moiety to ROS-generating cinnamaldehyde, which is therefore capable of amplifying oxidative stress in cancer cells to induce enhanced apoptotic cell death. The underlying hypothesis of the hybrid anticancer drug QCA is that depletion of antioxidant GSH by QM renders cancer cells more susceptible to cinnamaldehyde-mediated ROS insults and the elevated oxidative stress results in enhanced apoptotic cell death. In addition, QCA was designed to be activated by H 2 O 2 and acidic pH to release QM and cinnamaldehyde, respectively, in cancer environments and exert synergistic therapeutic actions. Herein, we demonstrate that the rationally designed hybrid drug QCA has dual mode of anticancer actions with synergistic therapeutic effects in the proof of concept studies in vitro as well as in vivo . Design and synthesis of QCA A hybrid anticancer drug QCA was designed to be activated by acidic pH and high level of H 2 O 2 (ref. 27 ). QCA as a dual stimuli-responsive hybrid anticancer agent was synthesized as shown in Supplementary Fig. 1 . First, QM-generating boronate compound 1 was synthesized from the reaction of 1,3-propanediol and (4-(hydroxymethyl)phenyl) boronic acid at room temperature for 2 days. 1 was obtained as a viscose colourless liquid and its chemical structure was confirmed by 1 H NMR ( Supplementary Fig. 2 ). Cinnamaldehyde was reacted with 2-(hydroxymethyl)-2-methylpropane-1,3-diol to give a cinnamaldehyde derivative 2 , which possesses an acid-cleavable acetal linkage. The presence of an acetal linkage in 2 was confirmed by the appearance of acetal protons at ∼ 5.1 p.p.m. ( Supplementary Fig. 3 ). 2 was then reacted with carbonyldiimidazole to give a cinnamaldehyde releasing compound 3 which is able to react with hydroxyl group of 1 . From a reaction of 1 and 3 , a hybrid anticancer drug QCA was obtained as a white solid. QCA was characterized by NMR and mass spectroscopy ( Supplementary Fig. 4 ). The acetal protons appeared at ∼ 5.1 p.p.m. and the methylene protons next to boronic ester appeared at ∼ 4.1 p.p.m., demonstrating the successful coupling of H 2 O 2 -responsive boronate to cinnamaldehyde via a carbonate linker. For comparison purposes, we also developed 4-(1,3,2-dioxaborinan-2-yl)benzyl benzyl carbonate, Q 1 , which is able to generate QM only in the presence of H 2 O 2 ( Supplementary Fig. 5 ), not cinnamaldehyde. Q 1 serves as a control to support the superior anticancer efficacy of QCA, which exerts synergistic effects of QM and cinnamaldehyde. Stimuli responsiveness of QCA It was reasoned that QCA rapidly undergoes H 2 O 2 -mediated boronate oxidation to release QM in accordance with the mechanism outlined in Supplementary Fig. 6 . In particular, the C–B bond is rapidly cleaved with the formation of 4 containing a phenol group, which exists in aqueous solutions in equilibrium with phenolate of 5 . The phenolate is known to rapidly undergo spontaneous 1,6-elimination with formation of QM that reacts with nucleophilic H 2 O to generate hydroxybenzyl alcohol [20] . We studied the dual stimuli-triggered activation of QCA by investigating NMR spectra after hydrolysis under tumour conditions ( Fig. 2a ). In the presence of 500 μM of H 2 O 2 , the generation of QM from QCA was indirectly confirmed by the appearance of aromatic proton peaks at ∼ 6.9 and ∼ 6.4 p.p.m. These observations are in good agreement with the previous studies reporting that QM is converted to hydroxybenzyl alcohol under aqueous conditions in the absence of nucleophiles such as GSH [7] , [28] , [29] , [30] . QCA also liberated cinnamaldehyde from the cleavage of acetal linkages after 48 h of incubation at acidic pH 6.5, confirmed by the reduced signal of acetal protons and appearance of aldehyde protons at 9.5 p.p.m. (ref. 23 ). It was determined that QCA undergoes H 2 O 2 -triggered hydrolysis with a second-order rate constant of 8.76 × 10 9 (lmol −1 s −1 ) and acid-triggered hydrolysis with a second-order rate constant of 3.24 × 10 3 (lmol −1 s −1 ). No changes were observed even after 72 h of incubation at neutral pH without H 2 O 2 , demonstrating that QCA is activated by only H 2 O 2 and acidic pH to generate cytotoxic QM and cinnamaldehyde, respectively. 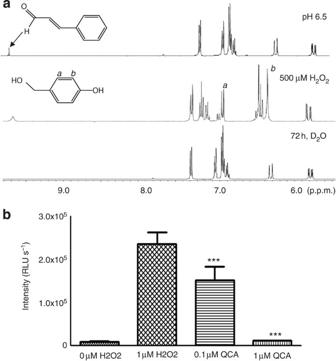Figure 2: Sensitivity of QCA to H2O2and pH. (a)1H NMR spectra of QCA before and after hydrolysis at acidic pH or in the presence of H2O2. (b) The sensitivity of QCA to H2O2assessed by peroxalate chemiluminescence. ***P<0.001 relative to a group of 1 μM H2O2(one-way analysis of variance,n=3, ±s.d.). RLU, relative light units. Figure 2: Sensitivity of QCA to H 2 O 2 and pH. ( a ) 1 H NMR spectra of QCA before and after hydrolysis at acidic pH or in the presence of H 2 O 2 . ( b ) The sensitivity of QCA to H 2 O 2 assessed by peroxalate chemiluminescence. *** P <0.001 relative to a group of 1 μM H 2 O 2 (one-way analysis of variance, n =3, ±s.d.). RLU, relative light units. Full size image The sensitivity of QCA to H 2 O 2 was also studied by measuring the level of H 2 O 2 based on peroxalate chemiluminescence, which has been used as a versatile tool for the detection of a variety of chemical species including fluorescent molecules and H 2 O 2 (refs 31 , 32 ). H 2 O 2 solution (1 μM) showed remarkably high emission intensity ( ∼ 1.1 × 10 5 relative light units) in the presence of fluorescent molecules and peroxalate ester ( Fig. 2b ). However, the addition of QCA to H 2 O 2 solution resulted in rapid and significant reduction in chemiluminescence intensity, concentration dependently. The majority of H 2 O 2 was rapidly reacted with the same concentration of QCA (1 μM) within 1 min. These observations suggest that the boronic ester in QCA specifically and quickly reacts with H 2 O 2 , resulting in the activation of QCA to release QM. Anticancer activity in vitro of QCA We first performed liquid chromatography–mass spectrometry (LC-MS/MS) analysis to confirm the generation of QM and cinnamladehyde in cells. The generation of QM from QCA was indirectly confirmed by measuring the level of cellular GSH, because it is impossible to detect QM that is an intermediate and rapidly reacts with nucleophilic GSH [7] , [20] . As shown in Supplementary Fig. 7 , lysates of DU145 cells treated with QCA for 24 h showed the remarkable (58%) reduction in the level of cellular GSH in comparison with untreated cells. QCA-treated cell lysates also showed a peak in LC trace identical to the standard cinnamaldehyde, while no peak was observed in untreated cell lysates. These findings clearly demonstrate that QCA generates both QM and cinnamaldehyde in cells. To further substantiate the depletion of antioxidant GSH by QCA, we investigated the effects of QCA on the level of GSH in various cells (prostate cancer DU145 cell line, colon cancer SW620 cell line and fibroblast NIH3T3 cell line). Cells were treated with various concentrations of QCA or Q 1 for 1.5 h and then the level of GSH was quantitatively measured using Ellman’s reagent as previously reported [7] . As shown in Fig. 3 , treatment of QCA or Q 1 resulted in significant reduction of the GSH level in malignant DU145 cells, in a dose-dependent manner. More than half of GSH was depleted in DU145 cells by both Q 1 and QCA at doses higher than 50 μM. QCA induced more GSH depletion in DU145 cells than SW620 cells. However, both QCA and Q 1 showed no effects on the GSH level in non-malignant NIH3T3 cells ( Supplementary Fig. 8 ). The above observations can be explained by the rationales that cancer cells have a greater extent of redox adaptation and malignant cells of different cancer types exhibit heterogeneity in the level of oxidative stress, associated with various expression of antioxidant systems [15] . It has been well known that metastatic prostate cancer cells including DU145 produce a large amount of ROS to have aggressive phenotypes [33] . However, cancer cells also generate a large amount of intrinsic antioxidants such as GSH, superoxide dismutase and catalase to counteract ROS and tolerate ROS-induced oxidative stress, leading to altered redox balance [1] , [17] . In particular, a large amount of GSH is known to play a critical role in cellular redox maintenance and antioxidative systems [8] , [10] . We also found that DU145 cells have the highest level of GSH and H 2 O 2 and the least level of GSH and H 2 O 2 were observed with normal NIH3T3 cells ( Supplementary Fig. 9 ). Therefore, rapid and remarkable reduction in the GSH level in prostate cancer DU145 cells was observed after the treatment of QCA, which rapidly generate QM. 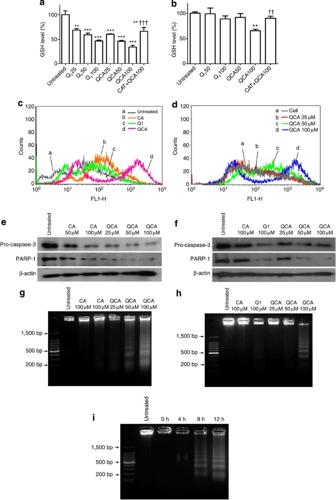Figure 3: Amplification of oxidative stress by QCA. Depletion of GSH by various concentrations of QCA and Q1in DU145 cells (a) and SW620 cells (b). The level of GSH was measured using Ellman’s reagents. The number indicates μM concentration. Catalase (CAT) was added to cells before the treatment of QCA. **P<0.01, ***P<0.001 relative to the untreated group,††P<0.01,†††P<0.001 relative to QCA 100 (one-way analysis of variance,n=4, ±s.d.), (c) ROS generation in DU145 cells treated with 100 μM of CA (cinnamaldehyde), Q1or QCA. (d) Concentration dependency of QCA on ROS generation in DU145 cells. For the detection of ROS, cells were stained with DCFH-DA and analysed using a BD FACSCaliber flow cytometer and CellQuest software. Cleavage of pro-apoptotic proteins in DU145 cells (e) and SW620 cells (f) as measured by Western blotting assay. Data are representative of four independent experiments. DNA fragmentation assay of DU145 cells (g) and SW620 cells (h) treated with various formulations for 12 h. (i) Time course of apoptosis of SW620 cells treated by 100 μm of QCA. Data are representative of three independent experiments. Figure 3: Amplification of oxidative stress by QCA. Depletion of GSH by various concentrations of QCA and Q 1 in DU145 cells ( a ) and SW620 cells ( b ). The level of GSH was measured using Ellman’s reagents. The number indicates μM concentration. Catalase (CAT) was added to cells before the treatment of QCA. ** P <0.01, *** P <0.001 relative to the untreated group, †† P <0.01, ††† P <0.001 relative to QCA 100 (one-way analysis of variance, n =4, ±s.d. ), ( c ) ROS generation in DU145 cells treated with 100 μM of CA (cinnamaldehyde), Q 1 or QCA. ( d ) Concentration dependency of QCA on ROS generation in DU145 cells. For the detection of ROS, cells were stained with DCFH-DA and analysed using a BD FACSCaliber flow cytometer and CellQuest software. Cleavage of pro-apoptotic proteins in DU145 cells ( e ) and SW620 cells ( f ) as measured by Western blotting assay. Data are representative of four independent experiments. DNA fragmentation assay of DU145 cells ( g ) and SW620 cells ( h ) treated with various formulations for 12 h. ( i ) Time course of apoptosis of SW620 cells treated by 100 μm of QCA. Data are representative of three independent experiments. Full size image In addition, GSH depletion in DU145 cells was significantly inhibited by the addition of H 2 O 2 -scavenging catalase, suggesting that the generation of QM from QCA is triggered specifically by H 2 O 2 . In the presence of catalase, QCA is unable to undergo H 2 O 2 -triggered boronate oxidation, resulting in no generation of GSH-depleting QM. More GSH depletion in DU145 cells than SW620 cells can also be explained by the more QM generation through H 2 O 2 -triggered boronate oxidation of QCA in DU145 cells, which has a larger amount of H 2 O 2 . Therefore, we envision that QCA has a tremendous potential for treating cancer cells that have a high extent of redox adaptation with a large amount of H 2 O 2 . The ability of QCA to induce ROS generation in cancer cells was studied by flow cytometry and confocal laser scanning microscopy. Cells were treated with free cinnamaldehyde, Q 1 or QCA and the level of ROS was measured using DCFH-DA (dichlorofluorescein-diacetate) as a fluorescent probe for intracellular ROS. After a short duration of treatment (12 h), free cinnamaldehyde (100 μM) slightly increased the level of ROS in DU145 cells, unlike our previous studies reporting that cinnamaldehyde induced significant ROS generation in SW620 cells after 24 h of treatment [23] . It may be because that in DU145 cells that have altered redox status with a high level of ROS as well as antioxidant systems, cinnamaldehyde-induced ROS would be destroyed by the high level of antioxidants and the additional H 2 O 2 generation by cinnamaldehyde is negligible compared with the high intrinsic level of ROS after a short period of time (12 h). Moderate rightward shift of DCFH-DA fluorescence was observed with Q 1 , indicating that GSH depletion favours ROS accumulation, as expected from Fig. 3a . However, QCA showed a significant rightward shift of DCFH-DA fluorescence in a dose-dependent manner ( Fig. 3c,d ), demonstrating the remarkably enhanced intracellular ROS accumulation. We also found that QCA-induced ROS accumulation was significantly inhibited by the treatment of H 2 O 2 -degrading catalase, evidenced by no rightward shift of DCFH-DA fluorescence ( Supplementary Fig. 10a ). QCA-induced ROS generation was also further confirmed by fluorescence micrographs ( Supplementary Fig. 10b ). QCA induced a dose-dependent ROS generation and catalase effectively reduced the level of ROS, suggesting that cinnamaldehyde released from QCA causes the generation of ROS including mainly H 2 O 2 and QM generation is inhibited by catalase. From these observations, it can be reasoned that QCA rapidly depletes GSH to suppress antioxidant systems, promoting massive accumulation of oxidative stress caused by cinnamaldehyde-mediated ROS. These results support our hypothesis that a hybrid anticancer drug QCA produces not only GSH-depleting QM but also ROS-generating cinnamaldehyde and both compounds act in a concerted manner to enhance oxidative stress. We next investigated the cytotoxicity of QCA by MTT (3-(4,5-dimethylthiazol-2-yl)-2,5-diphenyltetrazolium bromide) assay ( Supplementary Fig. 11 ). Cinnamaldehyde showed a moderate level of dose-dependent cytotoxicity in both DU145 and SW620 cells after 24 h of treatment, but minimal cytotoxicity in normal NIH3T3 cells. Despite the generation of antioxidant GSH-scavenging QM and subsequent ROS accumulation, Q 1 showed moderate cytotoxicity to cancer cells. The moderate cytotoxicity of QM-generating Q 1 is in agreement with previous studies which report that the sensitivity of the cancer cells towards cell death by QM is increased by pretreatment with a GSH-synthesis inhibitor ( L -buthionine-sulfoximine) [7] . However, a hybrid drug QCA exhibited a significantly higher cytotoxicity than cinnamaldehyde and Q 1 , which supports our hypothesis that GSH depletion by QM makes cancer cells more susceptible to ROS insults and subsequently ROS-generating cinnamaldehyde induces more cell death through amplified oxidative stress. It was also determined that QCA shows cytotoxicity with the half-maximal inhibitory concentration (IC 50 ) of 48 μM for DU145 cells and 76 μM for SW620 cells, but minimal cytotoxicity in normal NIH3T3 cells (IC 50 of 182 μM). We also found that co-treatment of catalase completely inhibited the cytotoxic effects of QCA, suggesting a strong relationship of QCA activity and H 2 O 2 . In the presence of H 2 O 2 -scavenging catalase, boronic ester groups of QCA cannot be cleaved, leading to no production of GSH-depleting QM, as aforementioned in Fig. 3 . Catalase also scavenges H 2 O 2 generated by cinnamaldehyde released from QCA. These findings clearly demonstrate that QCA exerts synergistic anticancer effects from sequential actions of antioxidant GSH-scavenging QM and ROS-generating cinnamaldehyde. To confirm whether QCA induces ROS-mediated apoptotic cell death, the expression of apoptosis-regulated proteins was investigated by the western blot assay. Figure 3e,f shows the effects of QCA on the expression of pro-apoptotic proteins, caspase-3 and poly(ADP ribose) polymerase (PARP), both critical enzymes involved in apoptosis. Cinnamaldehyde and QCA induced the cleavage of both pro-caspase-3 and PARP-1 in a dose-dependent manner ( Supplementary Fig. 12 ). However, QCA brought about a greater extent of cleavage of pro-caspase-3 and PARP-1, which confirms that QCA exerts superior apoptosis-inducing potential than cinnamaldehyde and Q 1 . We also studied the effects of QCA on DNA fragmentation, a hallmark of apoptosis ( Fig. 3g–i ). Cinnamaldehyde and Q 1 induced no or minimal DNA fragmentation. However, QCA-treated cells showed nucleosomal DNA fragmentation as clear DNA ladders of multiples of ∼ 180 bp, characteristics of apoptotic DNA fragmentation [34] . The amount of fragmented nucleosomal DNA gradually increased in concentration- and time-dependent manners. These observations demonstrate that QCA is capable of inducing apoptosis. The results of DNA fragmentation assay was further supported by the flow cytometric analysis using Annexin V-FITC (fluorescein isothiocyanate) as a marker of apoptosis and propidium iodide (PI) as a marker for cell viability. As shown in Supplementary Fig. 13 , QCA-treated cells showed greater populations of early apoptotic cells (in the lower right quadruple) and late apoptotic cells (in the upper right quadruple) than those treated with cinnamaldehyde and Q 1 . An increase in the population of Annexin V+and PI+cells was observed at higher dose of QCA. It is well known that ROS production and apoptosis are closely related and activation of caspase-3 is one of hallmark consequences of GSH depletion [35] , [36] . Therefore, the superior apoptosis-inducing potential of QCA is attributed to the combined effects of GSH-depleting QM and ROS-generating cinnamaldehyde. A mouse tumour xenograft model To investigate the in vivo anticancer activity of QCA, we used xenograft mouse models of SW620 and DU145 cells. Cancer cells were subcutaneously injected into the lower back of mice and dosing was initiated when small palpable tumours had developed. Various formulations (cinnamaldehyde, Q 1 , cinnamaldehyde along with Q 1 or QCA) were intravenously injected at a physiologically relevant dose of 2 mg kg −1 through a tail vein every 3 days. Mice inoculated with SW620 cells showed remarkable tumour growth for 22 days. Treatment of cinnamaldehyde alone or Q 1 alone showed marginal inhibitory effects on tumour growth at a dose of 2 mg kg −1 . The combined use of cinnamaldehyde with Q 1 also had moderate anticancer effects. However, mice treated with QCA developed significantly smaller tumour mass in comparison with the groups treated with cinnamaldehyde, Q 1 or the combination of cinnamaldehyde and Q 1 . At the same dose of 2 mg kg −1 , the superior anticancer actions of QCA over the combined use of cinnamaldehyde and Q 1 can be explained by the rationale that QCA could sequentially generate both QM and cinnamaldehyde in tumours, but free cinnamaldehyde has less ability to target tumours because of its low half-life in blood. To further evaluate the anticancer activity of QCA, tumour-bearing mice were treated with different doses of QCA, in comparison with commercial anticancer drug, camptotethin. Moderate anticancer effects were observed with QCA at doses <1 mg kg −1 , but remarkable anticancer effects at a dose of 2 mg kg −1 , comparable to camptotethin ( Fig. 4d ). Similar results were obtained using mice bearing DU145 tumour xenografts. Notably, marked antitumor effects were observed in mice treated with QCA at the same dose of 2 mg kg −1 ( Fig. 4g,h ). 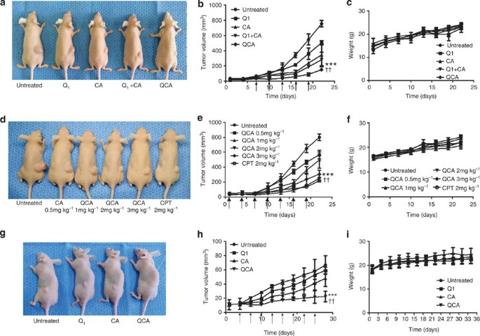Figure 4: Anticancer effects of QCA in mice inoculated with SW620 and DU145 cells. (a) Representative images of mice bearing SW620 tumour xenografts. Changes of tumour volumes (b) and body weight (c) in a SW620 xenograft model. ***P<0.001 relative to untreated,††P<0.01 relative to Q1+CA (one-way analysis of variance (ANOVA),n=4, ±s.d.). (d) Representative images of mice bearing SW620 tumour xenografts treated with various amounts of QCA and camptotethin (CPT). Changes of tumour volumes (e) and body weight (f) of mice bearing SW620 tumour xenografts during the treatment. ***P<0.001 relative to untreated,††P<0.01 relative to QCA 1 mg kg−1(one-way ANOVA,n=4, ±s.d.). (g) Representative images of mice bearing DU145 tumour xenografts. Changes of tumour volumes (h) and body weight (i) in a DU145 xenograft model. ***P<0.001 relative to untreated.††P<0.01 relative to CA (one-way ANOVA,n=4, ±s.d.). Arrows indicate the date of treatment. Figure 4: Anticancer effects of QCA in mice inoculated with SW620 and DU145 cells. ( a ) Representative images of mice bearing SW620 tumour xenografts. Changes of tumour volumes ( b ) and body weight ( c ) in a SW620 xenograft model. *** P <0.001 relative to untreated, †† P <0.01 relative to Q1+CA (one-way analysis of variance (ANOVA), n =4, ±s.d.). ( d ) Representative images of mice bearing SW620 tumour xenografts treated with various amounts of QCA and camptotethin (CPT). Changes of tumour volumes ( e ) and body weight ( f ) of mice bearing SW620 tumour xenografts during the treatment. *** P <0.001 relative to untreated, †† P <0.01 relative to QCA 1 mg kg −1 (one-way ANOVA, n =4, ±s.d.). ( g ) Representative images of mice bearing DU145 tumour xenografts. Changes of tumour volumes ( h ) and body weight ( i ) in a DU145 xenograft model. *** P <0.001 relative to untreated. †† P <0.01 relative to CA (one-way ANOVA, n =4, ±s.d.). Arrows indicate the date of treatment. Full size image We also performed LC-MS/MS analysis of tumour lysates at day 22 to confirm the generation of QM and cinnamaldehyde in tumours. As shown in Supplementary Fig. 14 , tumours of QCA-treated mice showed ∼ 38% less GSH level than those of untreated mice, indirectly supporting the generation of QM in tumours because QM rapidly reacts with nucleophilic GSH. The generation of cinnamaldehyde in tumours was also observed, as evidenced by the appearance of a new peak, identical to the standard cinnamaldehyde. However, QM and cinnamaldehyde were not detected in liver. These results demonstrate that QCA accumulates in tumours and generates both QM and cinnamaldehyde in tumour environments, leading to cancer cell death. The therapeutic efficacy of QCA was further confirmed by histological examination. Unlike tumour tissues from control mice consisting of abundant tumour cells with no obvious damages, tumours developed in QCA-treated mice had a large area of dead cells without nuclei ( Supplementary Fig. 15 ) [37] . In addition, QCA-induced apoptotic cell death was also confirmed by terminal deoxynucleotidyl transferase dUTP nick end labelling staining. QCA appeared well tolerated as judged by weight loss determination ( Fig. 4c,f,i ). QCA treatment also induced no notable tissue damages or lesions in liver and heart ( Supplementary Fig. 16 ). These observations clearly demonstrate potent anticancer activity of QCA, without severe system toxicity. Taken together, we envision that QCA is activated to produce both GSH-scavenging QM and ROS-generating cinnamaldehyde in cancer cells, which act in a synergistic fashion to kill cancer cells more specifically by amplifying the oxidative stress in a concerted manner. Finally, to test the safety profile of QCA, we administrated QCA (2 mg kg −1 ) into normal mice every other day for 10 days. QCA-treated mice showed no difference in the level of serum ALT (alanine transaminase) in comparison with untreated mice. In addition, there was no obvious histological evidence of accumulated toxicity in liver and heart associated with administration of QCA for 10 days ( Supplementary Fig. 17 ), demonstrating no or minimal toxicity of QCA. One of the major challenges in the development of anticancer therapeutic agents is the temporal and spatial therapeutic actions in a controlled manner [16] , [17] . There have been enormous efforts for the development of anticancer agents that are able to target specific oncogenic molecules to enhance therapeutic activities and specificity, by exploiting the genetic differences between normal cells and cancer cells. A prime example of selective anticancer drugs is imatinib (Gleevec, Norvatis), which targets the oncogenic tyrosine kinase BER-ABL responsible for myeloid leukaemia [17] , [38] . Despite the promising therapeutic activities and specificity, gene-targeting therapeutic strategies face challenges because of acquired drug resistance, genetic instability and multiple genetic alteration in cancer cells [16] . There are multiple lines of evidence indicating that cancer cells are under oxidative stress, reflecting altered redox balance. Cancer cells are more vulnerable to agents that impair redox balance and increase oxidative stress, but normal cells are less sensitive to the oxidative stress-inducing agents due to their low level of basal ROS and high antioxidant capacity. On the basis of the biochemical differences in cancer cells and normal cells, modulation of oxidative stress has recently been re-emerged as a therapeutic strategy to selectively target the destruction of cancer cells. Great efforts have been made for developing selective anticancer therapeutic agents that increase the level of ROS or alternatively suppress the antioxidant systems [1] , [12] , [16] , [33] , [39] , [40] , [41] . In this regard, we rationally designed a hybrid anticancer drug QCA to exploit oxidation therapy, which can not only increase the level of ROS but also weaken antioxidant systems simultaneously. We developed QCA that exerts dual and synergistic therapeutic actions in cancer environments associated with a high concentration of H 2 O 2 and acidic pH [8] , [27] . As shown in Fig. 1 , a hybrid anticancer drug QCA consists of an antioxidant GSH-scavenging moiety and ROS-generating cinnamaldehyde. QCA was also designed to have both H 2 O 2 -sensitive boronate and acid-sensitive acetal linkage. We confirmed that QCA rapidly undergoes H 2 O 2 -mediated oxidation to release QM, which is able to abrogate the key antioxidant GSH ( Fig. 2 ). In NMR analysis for H 2 O 2 -mediated degradation of QCA, QCA was treated with H 2 O 2 . In this study, the concentration of H 2 O 2 was 500 μM, which is much higher than its physiological concentration. However, the concentration of QCA was 15 mM, which is 30 times higher than the concentration of H 2 O 2 . It is therefore necessary to have sufficient amount (500 μM) of H 2 O 2 to react with a higher concentration (15 mM) of QCA and detect noticeable changes in NMR signal, as suggested in previous studies reporting the H 2 O 2 -mediated degradation of boronate compounds using high concentrations of H 2 O 2 such as 500 μM and even 500 mM (refs 30 , 42 , 43 ). Aryl boronate has been known to rapidly and selectively react with H 2 O 2 to generate QM, which alkylates antioxidant GSH, thus inhibiting the cellular antioxidant systems and triggering cell death [7] , [20] , [28] , [44] . It has been well accepted that the intracellular level of GSH is about <10 mM (refs 20 , 45 , 46 ). Interestingly, we found that 0.1 mM of QCA remarkably (> 60%) reduced the level of GSH ( Fig. 3a,b ). The remarkable GSH depletion by QCA can be explained by considering the elevated intracellular concentration of QCA after its cellular internalization. Hydrophobic QCA could easily penetrate into cells, as confirmed by LC-MS/MS data ( Supplementary Fig. 7 ). After cellular internalization, the intracellular concentration of QCA would be significantly increased by two to three orders of magnitude because the total amount of cytosol is much less than culture medium (that is, 1 ml in a well of 24-well plates). Therefore, QCA at a concentration of 0.1 mM in culture medium could deplete a majority of cellular GSH. These observations are in good accord with previous studies reporting that QM-generating drugs (0.1 mM) induced more than 50% reduction of cellular GSH level [7] . We also demonstrated that the inhibition of antioxidant GSH by QCA is attributed to rapid formation of QM from H 2 O 2 -mediated boronate oxidation ( Fig. 3a,b ). QCA also has an acetal linkage that degrades specifically in acidic tumour environments to release ROS-generating cinnamaldehyde. Simple treatment of cinnamaldehyde may not always lead to a preferential and sufficient killing of cancer cells. Depletion of cellular antioxidant GSH by QM would seem to be a logical approach in enhancing the anticancer potential of ROS-generating cinnamaldehyde [8] . Therefore, appealing features of rationally designed hybrid anticancer drug QCA are the dual stimuli responsiveness and sequential therapeutic actions, which results in synergistic anticancer effects in a cancer cell-specific manner. The results in proof of concept studies in vitro and further studies on mouse tumour xenograft models confirm the serial and synergistic anticancer activities of QCA. As illustrated in Fig. 1 , QCA not only suppresses antioxidant systems but also induces ROS generation, amplifying oxidative stress and leading to apoptotic cell death. Further optimization, including administration routes, dose, frequency, pharmacokinetics, pharmacodynamics, drug resistance studies and toxicology are warranted to maximize the full potential of QCA for clinical settings. In conclusion, we developed a dual stimuli-responsive anticancer hybdrid drug QCA that is activated by H 2 O 2 and acidic pH to generate antioxidant GSH-depleting QM and ROS-generating cinnamaldehyde, respectively, and amplifies oxidative stress to induce apoptotic cell death. Combination of QM and cinnamaldehyde displays a sequential mode of action in cancer treatment, by suppressing antioxidant systems and generating cytotoxic ROS in cancer cells specifically, further disturbing redox balance to kill cancer cells more effectively and specifically. To the best of our knowledge, the dual stimuli-responsive QCA is the first hybrid drug that not only inhibits antioxidant systems but also increases ROS stress simultaneously to kill cancer cells specifically. We anticipate that a novel hybrid drug QCA contributes to the development of new intelligent therapeutics based on the rational design of bioactive molecules and provides the best opportunities for efficient cancer treatment. Synthesis of (4-(1,3,2-dioxaborinan-2-yl)phenyl)methanol, 1 (4-Hydroxymethylphenyl) boronic acid (2.0 g) and 1,3-propanediol (1.0 g) were dissolved in 40 ml of dry tetrahydrofuran at room temperature. The reaction was allowed for 72 h with mechanical stirring. The solvent was evaporated and 1 was obtained using silica gel chromatography (hexane/ethyl acetate=6/4). Synthesis of cinnamaldehyde derivative 2 Tris(hydroxymethyl)ethane (4.88 g) was dissolved in 70 ml of dry benzene. Cinnamaldehyde (5.714 ml) and p -toluenesulfonic acid (40 mg) were added to the solution and the reaction was allowed for 4 h at 90 °C. After cooling the mixture to room temperature, 1 ml of triethylamine was added to terminate the reaction. Benzene was evaporated using a rotary evaporator and the product was obtained from column chromatography (hexane/ethyl acetate=7/3). Synthesis of cinnamaldehyde releasing compound 3 1,1′-Carbonyldiimidazole (4.1 g) and 2 (3.0 g) were dissolved in 50 ml of dry dichloromethane. The reaction was allowed for 30 min at room temperature. Dichloromethane was evaporated and the product was obtained from column chromatography using ethylacetate. Synthesis and characterization of QCA 1 (1.0 g) and 3 (1.7 g) were dissolved in 50 ml of dry dichloromethane containing 4-(dimethylamino)pyridine (0.64 g). The reaction was allowed for 24 h at 40 °C. After solvent evaporation, the product was obtained from column chromatography (hexane/ethyl acetate=5/5). QCA was characterized using NMR and GC–MS. 1 H NMR(400 MHz, CDCl 3 ): δ 7.2–7.8 (9H), 6.8 (1H), 6.2 (1H), 5.2 (1H), 5.1 (2H), 4.4(2H), 4.15 (4H), 4.0 (2H), 3.6(2H), 1.6 (2H), 0.85 (3H); 13 N NMR (400 MHz, CDCl 3 ): δ 155,5, 137.3, 135.9, 133.9, 133.7, 128.5, 128.5, 127.3, 126.8, 125.0, 101.1, 77.5, 77.3, 77.0, 72.7, 69.9, 33.8, 27.4, 17.0; LC-MS (m/z):[M] + calc. for C 25 H 29 O 7 B, 452.29; found 453.26; analysis (calcd., found for C 25 H 29 O 7 ): C (66.38, 65.44), H(6.46, 6.70). Sensitivity to H 2 O 2 The sensitivity of QCA to H 2 O 2 was evaluated by measuring the chemiluminescence intensity after the reaction with diphenyl oxalate solution including rubrene. QCA (0.1 or 1 μM) was added in the H 2 O 2 solution (1 μM). After 1 min reaction with H 2 O 2 , diphenyl oxalate solution was added to the H 2 O 2 solution, and the chemiluminescence intensity was measured by using a luminometer (Femtomaster FB 12, Zylux Corporation, TN, USA). Cellular GSH levels Cells (DU145, SW620 and NIH3T3) were obtained from Korean Cell Line Bank (Korea). Cells were seeded in a six-well plate (5 × 10 5 per well) and cultured to reach confluency of 80%. After treatment with various compounds for 1.5 h at 37 °C, cells were harvested, washed with PBS and then lysed on ice in 40 μl of Triton-X-100 lysis buffer. After 20 min, lysates were centrifuged at 9,800 g and 10 μl of the supernatant was mixed with 50 μl of Ellman’s reagent (0.5 mM DTNB). The amount of GSH was quantified by measuring the absorbance at 405 nm using a microplate reader (Biotek Instruments, Winooski, VT). Percentage of GSH content from treated cells were compared with basal GSH content measured in untreated cells. Flow cytometry DU145 or SW620 cells (4 × 10 5 ) were cultured in a 24-well culture plate for 24 h and treated with free cinnamaldehyde or QCA for 12 h. Cells were washed with fresh medium twice and resuspended in 1 × binding buffer at a concentration of 1 × 10 4 cells ml −1 . For the detection of ROS, the cell suspensions (1 ml) were transferred to a 5 ml culture tube and added with 5 μM of DCFH-DA (Sigma-Aldrich, St Louis, MO), followed by gentle mixing. The cells were incubated for 15 min at 37 °C in the dark and added with 400 μl of 1 × binding buffer. For the analysis of apoptosis, the cell suspensions were treated with Annexin V-FITC and propidium iodide (BD Biosciences Pharmigen, San Diego, CA). The stained cells were analysed by flow cytometry (FACS Caliber, Becton Dickinson, San Jose, CA). A total of 1.0 × 10 4 events were counted for each sample. Cytotoxicity of QCA The cytotoxicity of QCA was determined by MTT assay. DU145, SW620 cells and NIH3T3 cells were seeded at a density of 1 × 10 5 cells per well in a 24-well plate and incubated for 24 h to reach ∼ 90% confluency. Cells were treated with various amounts of QCA, Q 1 or cinnamaldehyde and incubated for 24 h. Each well was given 100 μl of MTT solution and were incubated for 4 h. The resulting formazan crystals were dissolved by 1 ml of dimethylsulfoxide. After 10 min of incubation, the absorbance at 570 nm was measured using a microplate reader (Biotek Instruments, Winooski, VT). The cell viability was determined by comparing the absorbance of QCA-treated cells to that of control cells. LC-MS/MS analysis of cell lysates Cells were seeded in a T-75 flask containing 10 ml of medium and allowed to attach for 24 h. Cells were treated with 100 μM of QCA or DMSO containing medium. After 24 h of incubation, cells were washed with new medium and cell pellets were added with 100 μl of methanol. The mixture was vortexed and then additional 900 μl of methanol was added. The contents were thoroughly mixed by vortexing and high molecular materials were removed by sequential centrifugation (10,000 g ) for 10 min. The supernatant was immediately stored at −80 °C until analysis. On analysis, 5 μl was injected and the peak for GSH and cinnamaldehyde was analysed using a LC-MS/MS spectrometer (6410 Triple Quad LC /MS/MS, Agilent Technologies, Willington) equipped with a column (Synergi 4 μ Hydro RP 80 A, 150 × 2.00 mm). Flow rate was 0.23 ml min −1 and the elution was with a gradient of water and acetonitrile (A= 0.1% Formic acid in water; B=0.1% Formic acid in acetonitrile): 0→1 min, 5% B; 1→10 min, 5% B; 10→14 min, 100% B, 14→20 min, 5% B). Detection was conducted at m/z 308→162.0 for GSH and m/z 133→114.9 for cinnamaldehyde. Ions were generated in positive ionization mode using electrospray ionization interface. The Fragmenter potential was set to 110 V and the interface heater was set to 300 °C. Immunoblot analysis DU145 cells (2 × 10 6 per well) or SW620 (1.7 × 10 6 per well) cells were treated with various concentrations of free cinnamaldehyde or QCA for 8 h and then washed with fresh PBS twice. Proteins were extracted from the cells using a lysis buffer. Electrophoresis was performed using 20 μg of cell lysate on a 10% polyacrylamide gel and proteins were transferred to PVDF membranes (Millipore, Billerica, MA). The blot was incubated with PARP monoclonal antibody (Santa Cruz Biotechnology, Dallas, TX) or caspase-3 (Santa Cruz Biotechnology, Dallas, TX) and HRP-conjugated anti-goat (Millipore, Billerica, MA), which is used as a secondary antibody. Immunoblot signals were developed using SuperSignal Ultra chemiluminescent reagent (Pierce, Rockford, IL). Images have been cropped for presentation. Full-size images are presented in Supplementary Fig. 12 . DNA fragmentation Cells (2 × 10 6 per well) cells were treated with various concentrations of free cinnamaldehyde or QCA for 12 h and then washed with fresh PBS twice. Chromosomal DNA was extracted from the apoptotic cells using Quick Apoptotic DNA Ladder Detection Kit (Life Technologies, Frederick, MD). In brief, the cells were lysed with TE buffer by pipetting up and down several times. The crude lysates were treated with enzyme solution until they became clear and mixed with ammonium acetate and ethanol. The mixtures were vortexed at −20 °C for 10 min to allow DNA to precipitate. The mixtures were centrifuged at 10,000 g to collect precipitated DNA. After careful removal of supernatant, DNA pellets were washed with 70% cold ethanol and recentrifuged at 10,000 g for 10 min. The supernatants were discarded and DNA was air dried at room temperature. DNA was then suspended with DNA Suspension Buffer by pipetting up and down several times. DNA was separated on agarose gel (1.8%), stained with ethidium bromide and photographed under ultraviolet light. Animal studies To evaluate the therapeutic efficacy of QCA, a subcutaneous tumour was established by inoculating SW620 cells (1.8 × 10 6 cells per mouse) or DU145 cells (2.0 × 10 6 cells per mouse), into the back of nude mice (male, 4 weeks, Orient Bio, Korea). When small palpable tumours had developed, the mice were randomly grouped and intravenously injected with one of the following: saline, Q 1 , cinnamaldehyde, cinnamaldehyde along with Q 1 or QCA through a tail vein. Each mouse was intravenously injected once every 3 days at a dose of 2 mg kg −1 . The body weight and tumour volume were recorded every 3 days. The length and width of the tumours were measured by digital calipers, calculating the tumour volume using the following formula: (width 2 × length)/2. At the end of the experiments, mice were killed and tumours were excised. Liver, heart and tumour tissues were histologically evaluated with haematoxylin and eosin staining. For LC-MS analysis, tumours were frozen in liquid nitrogen and ground into a fine power using a pestle and mortar. Tumour lysates were analysed using the same procedure for cell lysates. To evaluate the toxicity of QCA, QCA was injected into mice (male Balb/c of body weight of ∼ 20 g, Orient Bio, Korea) with QCA at a dose of 2 mg kg −1 every other day for 10 days. The activity of serum ALT was determined with an ALT enzymatic assay kit (Asan Pharma, Seoul, Korea) using a microplate reader (Synergy MX, BioTek Instruments Inc., Winooski, VT). The liver and heart tissues were fixed with 10% formalin (Sigma-Aldrich, St Louis, MO) and embedded into paraffin. Histological sections were made and stained with haematoxylin and eosin. All the animal experiments were carried out according to the guidelines of the institution animal ethical committee (CBU2014-00024). How to cite this article: Noh, J. et al . Amplification of oxidative stress by a dual stimuli-responsive hybrid drug enhances cancer cell death. Nat. Commun. 6:6907 doi: 10.1038/ncomms7907 (2015).